Ambient-stable tetragonal phase in silver nanostructures Crystallization of noble metal atoms usually leads to the highly symmetric face-centred cubic phase that represents the thermodynamically stable structure. Introducing defective microstructures into a metal crystal lattice may induce distortions to form non-face-centered cubic phases when the lateral dimensions of objects decrease down to nanometre scale. However, stable non-face-centered cubic phases have not been reported in noble metal nanoparticles. Here we report that a stable body-centred tetragonal phase is observed in silver nanoparticles with fivefold twinning even at ambient conditions. The body-centered tetragonal phase originates from the distortion of cubic silver lattices due to internal strains in the twinned nanoparticles. The lattice distortion in the centre of such a nanoparticle is larger than that in the surfaces, indicating that the nanoparticle is composed of a highly strained core encapsulated in a less-strained sheath that helps stabilize the strained core. Metal nanoparticles with tailored crystalline phases and internal microstructures (for example, twins and stacking faults) represent a class of promising building blocks in achieving ultrahigh-strength materials [1] , [2] , [3] , [4] , [5] , [6] , [7] , [8] and efficient catalysts [9] . Controlled synthesis of metal nanoparticles with well-defined compositions, sizes and morphologies has been extensively studied in the last decade [10] , [11] , [12] , [13] , [14] . However, noble metal nanoparticles with crystalline phases other than the closely packed face-centred cubic (f.c.c.) phase are rarely reported [15] , [16] . A body-centered tetragonal (b.c.t.) phase of silver (Ag) and other metals has been predicted by molecular dynamics simulations to be possible from a spontaneous phase transition of very thin f.c.c. nanowires (with diameters <2 nm) because of very high surface stresses in the nanowires [17] , [18] . The b.c.t. phase could also possibly exist in slightly thicker nanowires (with diameters <5 nm) by applying external high pressures to the nanowires [19] . Similar thickness-induced phase transitions have also been observed in ultrathin gold films and wires, but only for samples with lateral dimensions <2 nm [20] , [21] . However, Ag nanowires with such small diameters and b.c.t. phase have not been successfully synthesized due to their high surface energy and structural instability. On the other hand, we have observed that Ag nanoplates with multiple parallel twin planes exhibited a partial phase transition from f.c.c. to b.c.t. under external pressures higher than 12 GPa, although Ag nanocubes without internal crystalline defects remain perfect f.c.c. phase at even higher pressures [22] . These results indicate that controlling internal microstructures in nanoparticles may represent a promising strategy to achieve tetragonal phase even for nanoparticles with large lateral dimensions (for example, >10 nm) at ambient pressure. Here we report that a stable and pure b.c.t. phase exists in silver nanoparticles with fivefold twinning even in ambient environments. The b.c.t. phase originates from the distortion of cubic silver lattices due to internal strains in the twinned nanoparticles. The lattice distortion in the centre of such a nanoparticle is larger than that in the surfaces, indicating that the nanoparticle is composed of a highly strained core encapsulated in a less-strained sheath. The sheath can help the strained core to maintain large stresses and lattice distortion, resulting in an enhanced stability of the b.c.t. phase. These discoveries shed light onto the critical role of internal microstructures in determining properties of materials. Geometric structure of silver nanowires Silver nanowires ( Fig. 1a ) with a fivefold twinning structure have been synthesized through a modified polyol process, in which ethylene glycol reduces silver nitrate (AgNO 3 ) at elevated temperatures [23] . The nanowires exhibit an average diameter of 85 nm and pentagonal cross-sections (inset, Fig. 1a ). The unique fivefold symmetry is due to the existence of five {111} twin planes that cross along a line in the centre of each nanowire. Accordingly, each nanowire could be considered to be composed of five single-crystalline f.c.c. subunits sharing their {111} crystallographic faces ( Fig. 1b ). However, the five subunits cannot completely fill space as predicted by the simple solid-geometry model, leading to the formation of a solid-angle deficiency (inset, Fig. 1b ). This deficiency leads to lattice strains and/or defects in the synthesized nanowires to fill the 7.35° gap. In addition to Ag, the fivefold twinning represents a common structure in nanowires made of different coinage metals, such as Cu [24] and Au [25] . Although small multiply twinned nanoparticles (with sizes <5 nm) have been documented through transmission electron microscopy (TEM) and electron diffraction (ED) [26] , [27] , the proposed models for their existence cannot explain the stability of the fivefold metal nanowires with diameters >50 nm. 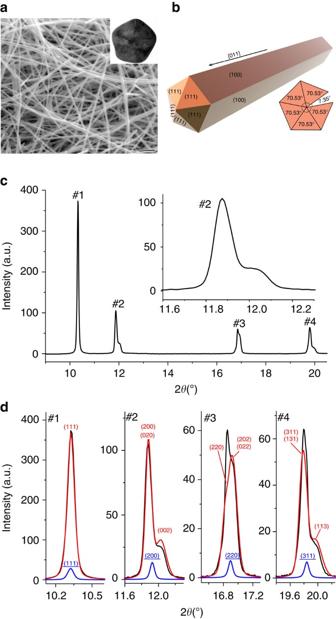Figure 1: Electron microscopy images and high-resolution X-ray diffraction patterns of Ag nanowires. (a) Scanning electron microscopy image of the Ag nanowires randomly assembled on the surface of a silicon wafer. The inset is a transmission electron microscopy image of the cross-section of a nanowire that was viewed parallel to the longitudinal axis of the nanowire. (b) Schematic drawing of a Ag nanowire with a fivefold symmetry. The surfaces and growth direction were indexed according to the electron diffraction patterns inFig. 2. (c) X-ray diffraction pattern of dried Ag nanowires obtained using an X-ray beam with a wavelength of 0.42460 Å. The inset highlights the splitting of the second peak. (d) Plots of the experimental X-ray diffraction pattern (black curves) and the fitted patterns against a face-centred tetragonal (f.c.t.) phase (red curves) and a face-centred cubic (f.c.c.) phase (blue curves). The f.c.t. fitting was plotted in the full scale, while the f.c.c. fitting plotted in a scale divided by 10. The peaks were indexed according to the standard f.c.t. and f.c.c. phase, respectively. The peak numbers are consistent incandd. The scale bar inarepresents 500 nm. a.u., arbitrary unit. Figure 1: Electron microscopy images and high-resolution X-ray diffraction patterns of Ag nanowires. ( a ) Scanning electron microscopy image of the Ag nanowires randomly assembled on the surface of a silicon wafer. The inset is a transmission electron microscopy image of the cross-section of a nanowire that was viewed parallel to the longitudinal axis of the nanowire. ( b ) Schematic drawing of a Ag nanowire with a fivefold symmetry. The surfaces and growth direction were indexed according to the electron diffraction patterns in Fig. 2 . ( c ) X-ray diffraction pattern of dried Ag nanowires obtained using an X-ray beam with a wavelength of 0.42460 Å. The inset highlights the splitting of the second peak. ( d ) Plots of the experimental X-ray diffraction pattern (black curves) and the fitted patterns against a face-centred tetragonal (f.c.t.) phase (red curves) and a face-centred cubic (f.c.c.) phase (blue curves). The f.c.t. fitting was plotted in the full scale, while the f.c.c. fitting plotted in a scale divided by 10. The peaks were indexed according to the standard f.c.t. and f.c.c. phase, respectively. The peak numbers are consistent in c and d . The scale bar in a represents 500 nm. a.u., arbitrary unit. Full size image Fivefold twinned nanowires are very complicated due to their unique geometry and twin planes. Experiments and atomistic simulations have shown that the fivefold twinning dramatically changes the mechanical properties (in terms of yield strength, ductility and so on) in comparison with Ag nanowires without twin planes [7] , [8] . Recently, Johnson et al . [28] analysed strain distributions (including both lattice-rotation distribution and shear-strain distribution) in a decahedral Au nanoparticles with a diameter of 17 nm, based on aberration-corrected high-resolution transmission electron microscopy (HRTEM). However, the influence of the internal strains on the crystallographic phase of these nanostructures was not studied. In this work, high-resolution X-ray diffraction (XRD), HRTEM and nanodiffraction were used to show for the first time the existence of an ambient-stable b.c.t. phase in Ag nanowires ( Fig. 1a ). Study of Ag nanostructures with XRD High-resolution XRD pattern ( Fig. 1c ) of the Ag nanowires exhibits major peaks close to those of the f.c.c. Ag (blue curves, Fig. 1d ), but with noticeable peak splitting not expected for the f.c.c. phase. Fitting the XRD data according to a b.c.t. phase with a bct = b bct =2.899 Å and c bct =4.058 Å (red curves, Fig. 1d ) accurately accounts for all reflections in the pattern, except the relative intensity between the subpeaks of peak #3. In the following discussion, a face-centred tetragonal (f.c.t.) Ag phase, in which each unit cell consists of two b.c.t. unit cells, is used for simplicity to compare with the most stable f.c.c. phase. In such an f.c.t. cell, the lattice parameters, a fct , b fct and c fct are 4.100, 4.100 and 4.058 Å, respectively, with ( c/a ) fct =0.9898, indicating that the fivefold twinning induces anisotropic stresses along different crystallographic axes. Meanwhile, the anisotropic distortion slightly compresses the f.c.t. unit cells by 0.22% ( V fct =68.215 Å 3 versus V fcc =68.368 Å 3 ) in comparison with the standard f.c.c. unit cells ( a fcc = b fcc = c fcc =4.089 Å as shown by the blue curves in Fig. 1d ). The f.c.t. phase remains stable for the Ag nanowires sandwiched between Kapton tapes that prevent the nanowires from being oxidized with air even after they have been stored at ambient environment for more than 2 years. The Ag nanowires dispersed in liquid solutions also exhibit the same tetragonal phase ( Supplementary Fig. S1 ), implying that the f.c.t. phase does not originate from drying of the nanowires. The minor discrepancy between the measured XRD pattern and the fitted pattern for the peak #3 in Fig. 1d is due to the high morphological anisotropy of the Ag nanowires. The longitudinal axis of each nanowire is along the [011] crystalline direction. When the dry silver nanowires are deposited on a substrate, the orientations of all the {110} planes cannot be equally distributed due to the high aspect ratios of the nanowires. As a result, the relative intensities of the (220), (202), (022) reflections exhibit variations in comparison with the standard powder diffraction pattern. On the other hand, the Ag nanowires dispersed in a liquid solution randomly orient along different directions, leading to a diffraction pattern consistent with the standard pattern ( Supplementary Fig. S1 ). In addition, the f.c.t. phase is observed in different Ag nanowires with varying diameters that are synthesized via different synthetic strategies ( Supplementary Fig. S2 ). Moreover, decahedral Ag nanoparticles ( Fig. 2a ) with fivefold twin planes (highlighted by the red strips in Fig. 2b ) also exhibit an f.c.t. phase. The splitting between (200)/(020) and (002) peaks is weaker than the Ag nanowires ( Fig. 2c ). Owing to the less morphological anisotropy, the relative intensities of (200)/(020) and (002) peaks are consistent with the standard XRD pattern of f.c.t. Ag. In contrast, single-crystalline, defect-free Ag nanocubes ( Supplementary Fig. S3 ) exhibit perfect f.c.c. phases ( Supplementary Fig. S4 ) regardless of their sizes. The difference of crystalline phases ( Supplementary Fig. S5 ) in different nanoparticles confirms that the fivefold twinning structure can induce strong lattice strains responsible for the tetragonal distortions. 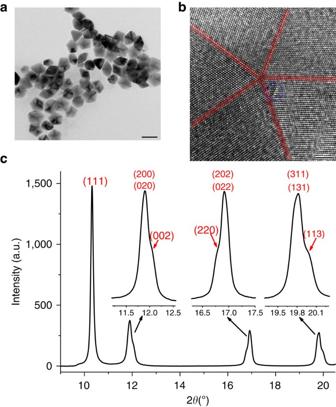Figure 2: Transmission electron microscopy (TEM) images and X-ray diffraction pattern of decahedral Ag nanoparticles. (a) TEM image of nanoparticles randomly assembled on a TEM grid. (b) High-resolution TEM image taken from the centre of an individual nanoparticle by aligning the electron beam parallel to the common axis of the five subunits of the nanoparticle. The red lines highlight the existence of five twin planes that cross along the common axis. Crystalline defects highlighted in the circle can be observed in this image, although the number of defects is less than that of the Ag nanowires shown inFig. 3f. (c) High-resolution X-ray diffraction pattern obtained from dried nanoparticles at room temperature with the use of an X-ray beam having a wavelength of 0.42460 Å. The peaks are indexed according to a face-centred tetragonal (f.c.t.) phase of Ag. The scale bars inaandbrepresent 50 and 2 nm, respectively. a.u., arbitrary unit. Figure 2: Transmission electron microscopy (TEM) images and X-ray diffraction pattern of decahedral Ag nanoparticles. ( a ) TEM image of nanoparticles randomly assembled on a TEM grid. ( b ) High-resolution TEM image taken from the centre of an individual nanoparticle by aligning the electron beam parallel to the common axis of the five subunits of the nanoparticle. The red lines highlight the existence of five twin planes that cross along the common axis. Crystalline defects highlighted in the circle can be observed in this image, although the number of defects is less than that of the Ag nanowires shown in Fig. 3f . ( c ) High-resolution X-ray diffraction pattern obtained from dried nanoparticles at room temperature with the use of an X-ray beam having a wavelength of 0.42460 Å. The peaks are indexed according to a face-centred tetragonal (f.c.t.) phase of Ag. The scale bars in a and b represent 50 and 2 nm, respectively. a.u., arbitrary unit. Full size image Study of Ag nanostructures with electron microscopy As highlighted by the circle in Fig. 2b , lattice strain in the Ag decahedral nanoparticles is large enough to induce the formation of lattice defects in the centre of the nanoparticles. More lattice defects are expected to exist in the Ag nanowires ( Fig. 1a ) because of larger lattice strains in the Ag nanowires than that in the decahedral Ag nanoparticles ( Fig. 2a ). As the five subunits merge together in each nanowire, simply rotating the nanowires on a TEM grid cannot allow us to appropriately align the electron beam for analysing individual subunits ( Supplementary Fig. S6 ). Therefore, we have sliced the nanowires to expose appropriate crystallographic surfaces by using focused ion beam (FIB) technique. 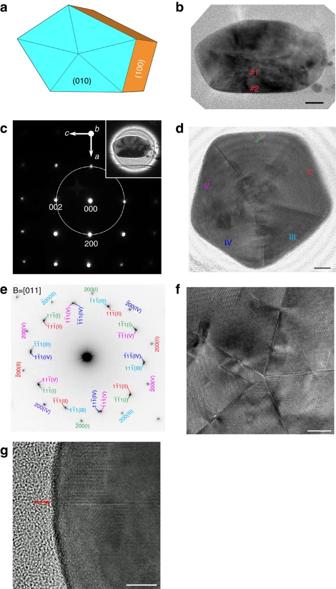Figure 3: Transmission electron microscopy images and electron diffraction patterns of different cross-sections of individual Ag nanowires. (a–c) Cross-section obtained by slicing a nanowire against the planes that have 45° with respect to the longitudinal axis of the nanowire. The inset incpresents a shadow image with the strongest contrast in the bottom subunit, indicating that the electron beam was well aligned against the low-index crystallographic axis of <010>. The electron diffraction (ED) pattern incwas recorded from the point #1 inbwith an electron beam of ~10 nm in size. The reflection spots were indexed according to the difference ofd-spacing along different crystallographic axes. The white circle whose centre overlaps the (000) reflection spot clearly shows that the (002) reflection spot is slightly farther than the (200) spot from the pattern centre, that is, the (000) spot. (d–g) Cross-section obtained by cutting a nanowire against the planes that are perpendicular to the longitudinal axis of the nanowire. The colours and Roman numerals in the parentheses correspond to the individual subunits labelled with the same colours and Roman numerals ind. The red arrow inghighlights the twin plane. The scale bars inbanddrepresent 20 and 10 nm, respectively. The scale bars in bothfandgrepresent 5 nm. Figure 3a,b present the schematic drawing and TEM image of a portion of a nanowire obtained by cutting the nanowire along the surfaces with an angle of 45° with respect to the longitudinal axis of the nanowire ( Supplementary Fig. S7 ). This cutting exposes one of the {100} surfaces in the bottom subunit. The ED pattern obtained from the position #1 ( Fig. 3b ) exhibits a rectangular symmetry showing a difference of 3.6%(±0.6%) between the d -spacing (that is, interplanar distance) of the (200) and (002) reflections ( Fig. 3c ). The non-uniform d -spacing along different <100> directions is consistent with the f.c.t. phase of the Ag nanowires. The difference significantly decreases to 0.8%(±0.6%) for position #2 that is located closer to the periphery of the nanowire ( Fig. 3b ), indicating that the lattice strains are concentrated in the central region. Figure 3: Transmission electron microscopy images and electron diffraction patterns of different cross-sections of individual Ag nanowires. ( a – c ) Cross-section obtained by slicing a nanowire against the planes that have 45° with respect to the longitudinal axis of the nanowire. The inset in c presents a shadow image with the strongest contrast in the bottom subunit, indicating that the electron beam was well aligned against the low-index crystallographic axis of <010>. The electron diffraction (ED) pattern in c was recorded from the point #1 in b with an electron beam of ~10 nm in size. The reflection spots were indexed according to the difference of d -spacing along different crystallographic axes. The white circle whose centre overlaps the (000) reflection spot clearly shows that the (002) reflection spot is slightly farther than the (200) spot from the pattern centre, that is, the (000) spot. ( d – g ) Cross-section obtained by cutting a nanowire against the planes that are perpendicular to the longitudinal axis of the nanowire. The colours and Roman numerals in the parentheses correspond to the individual subunits labelled with the same colours and Roman numerals in d . The red arrow in g highlights the twin plane. The scale bars in b and d represent 20 and 10 nm, respectively. The scale bars in both f and g represent 5 nm. Full size image As discussed previously, the lattice strains and distortions originate from the constraint of matching adjacent subunits against the {111} twin planes. It is important to analyse the microstructures near the twin planes in the cross-sectional sample shown in Fig. 3d . Aligning the electron beam parallel to the common axis of the five subunits (that is, the [011] crystallographic direction) results in a complex ED pattern ( Fig. 3e ). The reflections exhibit an approximately fivefold symmetry that is consistent with the geometry of the cross-section. However, the (111) reflections from two adjacent subunits are not merged into single symmetric spots ( Fig. 3e and Supplementary Fig. S8 ). The splitting of the (111) reflections indicates that the solid-angle gaps between the adjacent subunits are not filled with continuous lattices. The solid-angle gaps induce lattice defects, including stacking faults, associated partial dislocations, slips and possible additional small crystal domains, as shown in the HRTEM image of the centre ( Fig. 3f ). These defects are responsible for partially alleviating the strong internal strains to stabilize the f.c.t. nanowires. In contrast, the crystalline lattices near surfaces are essentially free of defects, except the {111} twinning plane ( Fig. 3g ), potentially indicating much less strain in the surface regions ( Supplementary Fig. S9 ). Cross-sectional samples of different nanowires ( Supplementary Fig. S10 ) exhibit the similar morphology and microstructures ( Supplementary Fig. S11 ), indicating that each Ag nanowire is a core/shell structure with a strained core that is responsible for the f.c.t. phase and a thin less-strained sheath that protects the core. Real-time probing of removal of cores in Ag nanowires The Ag nanowires can react with an aqueous solution of HAuCl 4 through a galvanic replacement reaction, leading to the formation of epitaxial Ag–Au alloy nanotubes ( Supplementary Fig. S12a ) [29] , [30] . The resulting nanotubes maintain the pentagonal cross-section of the Ag nanowires and also have fivefold twin planes that do not cross ( Supplementary Fig. S12b ). We have used time-resolved high-energy synchrotron X-ray diffraction to monitor in real-time the variation of the crystalline phase of the Ag nanowires during the reaction ( Supplementary Fig. S13 ). As the reaction proceeds, the characteristic double peaks of f.c.t. Ag near d ≈2.0 Å gradually disappear and eventually merge together to form a single peak corresponding to f.c.c. Ag–Au alloy ( Fig. 4 ). The compositional change from pure Ag to Ag/Au alloy is not responsible for the variation of XRD patterns because both unstrained, pure Ag and Au crystals exhibit the same f.c.c. phase and have very similar lattice constants (4.0862 and 4.0786 Å for Ag and Au, respectively) [31] . Hence, the change of crystalline structure from f.c.t. to f.c.c. phase well agrees the morphological variation from solid nanowires to hollow nanotubes. Owing to the absence of solid core, the five twin planes in each nanotube cannot cross and thus the strained tetragonal phase cannot be maintained, leading to an undistorted f.c.c. lattice. These results confirm that the core/shell structure of the Ag nanowires and the high strains associated with the tetragonal distortion are stored in the solid cores. 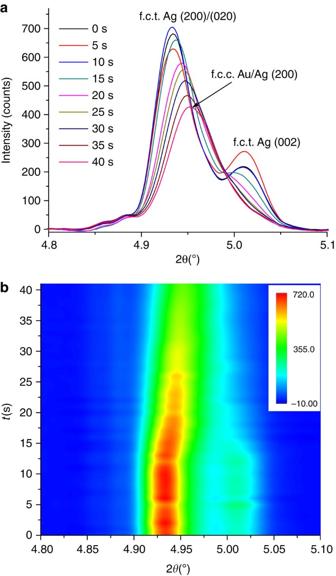Figure 4: Time-dependent synchrotron high-energy XRD patterns of the Ag nanowires during their transformation to hollow Ag–Au alloy nanotubes. (a) X-ray diffraction patterns plotted with a time interval of 5 s. (b) Contour plot of the diffraction patterns with a time interval of 1 s. The background caused by the solvent was subtracted for visual clarity. The wavelength of the X-ray beam was 0.1771 Å. Figure 4: Time-dependent synchrotron high-energy XRD patterns of the Ag nanowires during their transformation to hollow Ag–Au alloy nanotubes. ( a ) X-ray diffraction patterns plotted with a time interval of 5 s. ( b ) Contour plot of the diffraction patterns with a time interval of 1 s. The background caused by the solvent was subtracted for visual clarity. The wavelength of the X-ray beam was 0.1771 Å. Full size image From the experimental observations, it is concluded that a stable tetragonal crystalline phase exists in Ag nanoparticles under ambient environments. A fivefold twinning structure is key to the formation and stability of this tetragonal phase. This discovery underscores the importance of internal microstructures of nanoparticles in determining their crystalline phases and properties, although this relationship is often ignored. Both in situ and ex situ studies reveal that each Ag nanowire is composed of a heavily strained core and a less-strained sheath. The core/shell structure is responsible for the enhanced stability of the f.c.t. phase in the Ag nanowires and the strong driving force for their anisotropic growth. This discovery sheds the light on that the internal structures may have a more deterministic role in the growth of nanoparticles with controlled morphologies and tailored properties in comparison with external chemical environments. For example, in the well-determined core/shell Ag nanowires the cores are continuous along their longitudinal axes and exposed only at the ends of the nanowire ( Supplementary Fig. S14 ). The crystalline defects where the cores are exposed provide active sites for growing the nanowires along their longitudinal axes, while the less-strained side surfaces of the nanowires have lower reactivity towards the deposition of silver atoms for growing them thicker. The different reactivity between the end surfaces and side surfaces of the nanowires may be the major driving force for anisotropic growth of the nanowires. Synthesis of Ag nanowires Silver nanowires were synthesized through a modified polyol process reported elsewhere [23] . In a typical synthesis, 5 ml of ethylene glycol (J.T. Baker) was added to a 100-ml three-neck round flask, which was partially immersed in an oil bath setting at 160 °C. Heating was then continued under ambient pressure for 1.5 h. Meanwhile, solutions of AgNO 3 (0.10 M, Aldrich) and poly(vinyl pyrrolidone) (PVP, M W =55,000, Aldrich, 0.15 M, the concentration was calculated in terms of the repeating unit) were prepared by dissolving appropriate amount of AgNO 3 and PVP powders in 10 ml of ethylene glycol at room temperature with stirring. To 10 ml of PVP solution were added 22 μl of 100 mM NaCl (Fisher) solution and 200 μl of 0.5 mM tris(acetylacetonato)iron(III) (Fe(acac) 3 , Aldrich) solution, resulting in final concentrations of 0.06 mM and 2.2 μM for NaCl and Fe(acac) 3 , respectively. In the next step, 3 ml of each solution (that is, AgNO 3 and PVP with additives) were simultaneously delivered into the hot ethylene glycol with a syringe pump (KDS-200, KD Scientific, Holliston, MA) at a rate of 45 ml h −1 . The reaction was maintained at 160 °C for additional 1.5 h. Finally, the flask was removed from the oil bath to cool the resulting dispersion of Ag nanowires to room temperature. Magnetic stirring at 240 r.p.m. was applied throughout the entire synthesis. Synthesis of decahedral Ag nanoparticles Silver nanoparticles with decahedral morphology were synthesized by following a photochemical conversion strategy reported in literature [32] . In a typical synthesis, a precursor dispersion of very small Ag nanoparticles was first prepared by reducing AgNO 3 (Sigma-Aldrich) with NaBH 4 (Sigma-Aldrich) in an aqueous solution. To a 7.0 ml of deionized water in a 20-ml glass vial (VWR) were added 0.5 ml of 50 mM sodium citrate (Fisher), 0.015 ml of 50 mM PVP, 0.05 ml of 5 mM L -arginine (Sigma-Aldrich), and 0.2 ml of 5 mM AgNO 3 aqueous solutions. Addition of 0.08 ml of 0.1 M NaBH 4 aqueous solution freshly prepared right before the experiment to the above solution quickly reduced AgNO 3 . The solution became bright yellow after the reaction lasted for 10 min under a magnetic stirring at 250 r.p.m., indicating the formation of small Ag nanoparticles. The yellow solution of precursor Ag nanoparticles was then exposed to a 400-W metal halide lamp (Sunmaster, OH) to photochemically transform the precursor Ag nanoparticles into decahedral nanoparticles. Illuminating the precursor solution for 5 h led to a colour change from bright yellow to a red/green bicoloured appearance, indicating the formation of decahedral Ag nanoparticles. Synthesis of Ag nanocubes Silver nanocubes with an average size of 35 nm were synthesized by following the fast-injection method we developed previously [33] . In a typical synthesis, 8.0 ml of octyl ether (OE, 99%, Sigma-Aldrich) and 1.0 ml of oleylamine (OAm, assay 70%, primary amine >98%, Sigma-Aldrich) were added to a 50-ml three-neck flask connected to a Schlenk line that was purged with nitrogen. Dimethyldistearylammonium chloride (>97%, Sigma-Aldrich) powder (0.176 g or 0.3 mmol) was added to the binary solvent (OE–OAm) under strong magnetic stirring. The solvent was then heated to 60 °C by placing the flask on a heating mantle that was controlled by a digital thermal controller and the temperature was maintained for 10 min to completely dissolve dimethyldistearylammonium chloride. The resulting colourless solution was then quickly heated up to 260 °C. After the temperature was stabilized at 260 °C, 1.0 ml of an OAm solution of AgNO 3 (0.2 M) that was preheated at 50 °C was quickly injected into the flask with a syringe. Maintaining the reaction at 260 °C for 1 h completed the synthesis of Ag nanocubes. The reaction solution was then quickly cooled down to room temperature within 5 min by removing the heating mantle and blowing air to the surface of the reaction flask. Nitrogen purging and magnetic stirring (600 r.p.m.) were maintained throughout the entire synthesis. Silver nanocubes with size of ~120 nm were synthesized through a modified polyol process described in our previous work [29] . In a typical synthesis, 5 ml of anhydrous ethylene glycol (99.8%, Sigma-Aldrich) was heated in a 100-ml three-neck flask that was immersed in an oil bath setting at 160 °C for 1 h. A 3-ml aliquot of an ethylene glycol solution of 0.25 M AgNO 3 and a 3-ml aliquot of an ethylene glycol solution of 0.19 M PVP were simultaneously added to the hot ethylene glycol using a two-channel syringe pump at a rate of 0.375 ml min −1 . The reaction mixture was continuously heated at 160 °C for 40 min. Magnetic stirring (at a rate of 400 r.p.m.) was maintained throughout the synthesis. X-ray diffraction patterns of the Ag nanoparticles Dispersions of the as-synthesized Ag nanoparticles were centrifuged and rinsed with ethanol for three times followed by drying them under ambient environment. The dried nanoparticles were then transferred to Kapton tapes and sealed in the tapes for the synchrotron XRD measurements at the Advanced Photon Source. A Mar345 area detector was used to collect two-dimensional diffraction patterns, which were converted to one-dimensional curve of intensity as a function of 2 θ using the fit2d software. The detector was calibrated using a diffraction pattern of the CeO 2 standard powder sample. Preparation of cross-sectional samples of Ag nanowires A quantity of 0.1 ml of the original dispersion of the as-synthesized Ag nanowires was diluted with 0.9 ml ethanol followed by centrifuge at 4,000 r.p.m. for 10 min. The supernatant was discarded and the precipitate nanowires were then re-dispersed with 1 ml ethanol. Repeating centrifuge and re-dispersion for two more times. The resulting nanowires were then dispersed in 10 ml ethanol for sample preparation. One droplet of the dispersion was then placed on the carbon film (with thickness of 25 nm) of a TEM grid followed by evaporation of ethanol in a fume hood. Once ethanol was completely evaporated, the Ag nanowires attached to the surface of the carbon film. Site-specific cross-sectional samples were prepared with the use of a Zeiss cross-beam scanning electron microscope (SEM)/FIB (FIB–SEM) system with a gas injection system and micromanipulator in the Electron Microscopy Center at Argonne. To eliminate surface damage from the ion beam during sample preparation, the entire surface of the TEM grid with the Ag nanowires was coated with a layer of C (~50 nm thick) through thermal evaporation. The TEM grid was then loaded into the chamber of the FIB–SEM. A layer of Pt with thickness of ~100 nm was then deposited onto the C layer in the interested areas by using electron beam deposition (2 kV) associated with the in situ FIB gas injection system system. Another layer of Pt with thickness of ~300 nm was deposited using 30-kV ion beam deposition across the entire liftout bar. Both sides of the liftout bar were then cleaned with 30-kV ion beam milling. In the next step, the TEM grid was flipped over and layers of Pt with thickness of ~100 nm and C with thickness of 300 nm were sequentially deposited with the assistance of electron beam and 30-kV ion beam, respectively. The Ag nanowires in the resulting liftout bar were completely protected by the deposited Pt/C layers. Finally, a conventional FIB liftout method [34] was used to prepare the cross-sectional TEM samples. Once the liftout bar was thin enough (<100 nm) through 30-kV ion milling, a 5-kV ion beam was used to remove surface-damaged layers. Electron microscopic characterization A JEOL 2100F in the Center for Nanoscale Materials and the Argonne Chromatic Aberration-corrected TEM in the Electron Microscopy Center at Argonne were used to characterize both the as-synthesized Ag nanoparticles and the cross-sectional samples. Both TEMs were operated at an accelerating voltage of 200 kV. The bright field images, HRTEM images, EDs and nanodiffractions were recorded on the JEOL 2100F machine. HRTEM was carried out on Argonne Chromatic Aberration-corrected TEM. Real-time probing of galvanic reaction of Ag nanowires The reaction was probed with in situ time-resolved high-energy synchrotron XRD with the use of 70-keV ( λ =0.1771 Å) X-rays at 1-ID-C at Advanced Photon Source. The use of high-energy X-rays is advantageous for probing solution-phase reactions because of their strong penetration in liquid solvents and weak interactions with reactants. In a typical experiment, 1 ml dispersion of the Ag nanowires was added to a quartz cuvette (with an optical length of 10 mm) followed by heating the dispersion to 100 °C. Once the temperature was stabilized, the beamline hutch was closed and the X-ray beam was turned on. An aqueous solution of 0.1 M HAuCl 4 was then slowly injected to the hot dispersion of Ag nanowires to trigger the galvanic replacement reaction. Meanwhile, the XRD patterns were collected at a time interval of 1 s. How to cite this article : Sun Y. et al . Ambient-stable tetragonal phase in silver nanostructures. Nat. Commun. 3:971 doi: 10.1038/ncomms1963 (2012).